Linc-YY1promotes myogenic differentiation and muscle regeneration through an interaction with the transcription factor YY1 Little is known how lincRNAs are involved in skeletal myogenesis. Here we describe the discovery of Linc-YY1 from the promoter of the transcription factor (TF) Yin Yang 1 ( YY1 ) gene. We demonstrate that Linc-YY1 is dynamically regulated during myogenesis in vitro and in vivo . Gain or loss of function of Linc-YY1 in C2C12 myoblasts or muscle satellite cells alters myogenic differentiation and in injured muscles has an impact on the course of regeneration. Linc-YY1 interacts with YY1 through its middle domain, to evict YY1/Polycomb repressive complex (PRC2) from target promoters, thus activating the gene expression in trans . In addition, Linc-YY1 also regulates PRC2-independent function of YY1. Finally, we identify a human Linc-YY1 orthologue with conserved function and show that many human and mouse TF genes are associated with lincRNAs that may modulate their activity. Altogether, we show that Linc-YY1 regulates skeletal myogenesis and uncover a previously unappreciated mechanism of gene regulation by lincRNA. Normal skeletal muscle growth and the regeneration of damaged muscle fibres are attributed to satellite cells (SCs; muscle stem cells), which become immature muscle cells or myoblasts (MBs) and then proliferate and differentiate [1] . The differentiation stage is controlled by a complex network of muscle-specific transcription factors (TFs) including MyoD family, MEF2 family (MEF2A–D) and other general TFs [2] , [3] . Yin Yang 1 (YY1) is a ubiquitously expressed TF, which in proliferating MBs represses multiple muscle loci by recruiting histone methyltransferase Ezh2 (enhancer of zeste homologue 2) containing Polycomb repressive complex 2 (PRC2) [4] , [5] , [6] , [7] , [8] . When myogenesis ensues, YY1/PRC2 need to be removed and replaced by the MyoD/PCAF/SRF complex, leading to gene activation. The disengagement of YY1/PRC2 in a timely manner is thought to be induced by the degradation of the proteins [9] . However, a substantial reduction of the proteins was not observed until very late into terminal differentiation [6] , [9] , [10] , suggesting that alternative mechanisms may exist to ensure the effective removal of YY1/PRC2. Interestingly, we have recently discovered that in addition to PRC2-dependent repressive function on a small set of targets, YY1 possesses PRC2-independent function genome wide [11] . Nevertheless, YY1/PRC2 co-regulation of their target loci still exerts a pivotal role in myogenesis considering the importance of silencing them in MBs, thus warranting the further exploration of the molecular mechanism especially pertaining how YY1/PRC2 is removed from the targets on differentiation starts. Originally identified by Guttman et al. [12] using chromatin-state map, lincRNAs (large intergenic noncoding RNAs) are discrete transcriptional units intervening known protein-coding loci and they have quickly fuelled enthusiasm for research in the past few years. A combination of chromatin-state maps, RNA-sequencing (RNA-seq) data and computer algorithms was developed into a standard approach for de novo discovery of lincRNAs, which has led to cataloguing of lincRNAs with unprecedented speed in various organisms and cell types [13] . Owing to their cell-type specificity, there is little overlap between these catalogues, thus warranting the need for generating a muscle-specific catalogue. Recent work suggested various molecular mechanisms for lincRNAs and the current best characterized is in the regulation of epigenetic dynamics and gene expression [13] , [14] , [15] . A significant portion of functional lincRNAs are implicated in coordinating gene silencing pathways through direct interaction with repressive chromatin complexes such as PRC2 (refs 15 , 16 , 17 , 18 , 19 , 20 ). In recent times, examples of gene-activating lincRNAs are also emerging including HOTTIP [21] , ncRNA-a7 (ref. 22 ) and a large class of enhancer-associated long noncoding RNAs (lncRNAs) [23] . Divergent transcripts are a unique type of lincRNAs arising from bidirectional promoters of protein-coding genes. Increasing evidence indicates that promoters of protein-coding genes are origins of pervasive ncRNA transcription [24] , [25] , [26] . It is still debatable whether these divergent transcripts in general predominantly influence neighbouring ( cis ) or distal ( trans ) protein-coding genes. The known examples ( ncRNA-a1-7, Hottip, Mistral and so on) favour the prevalence of cis -acting function [13] , [27] despite many other observations challenging the notion that most lincRNAs work in cis [28] . However, examples to support the trans function are rare and the functional mechanisms are underexplored. In this study, we describe the discovery of Linc-YY1 , a divergently transcribed long noncoding transcript upstream of mouse YY1 -coding gene. The expression of Linc-YY1 is under control by MyoD and dynamically regulated in various settings of in vitro and in vivo myogenesis. During C2C12 and SC differentiation, its expression is induced and functionally promotes the differentiation programme. Loss of Linc-YY1 in injury-induced muscles delays the regeneration process. Mechanistically, Linc-YY1 binds YY1, leading to YY1/PRC2 eviction from target promoters and subsequent gene activation. In addition, genome-wide binding mapping also reveals putative function of Linc-YY1 in regulating YY1 activity independent of PRC2. Lastly, Linc-YY1 function is conserved in humans; moreover, many TFs in human and mouse are associated with divergently transcribed lincRNAs within their promoters, which may modulate their transcriptional activities. Altogether, we have identified and characterized a novel lincRNA involved in skeletal muscle cell differentiation and muscle regeneration. We have also elucidated a new mechanism through which divergently transcribed lincRNA modulates TF activity. Discovery of Linc-YY1 in myogenesis To generate a comprehensive catalogue of lincRNAs in muscle cells, we applied an integrated analysis on RNA-seq data generated by Trapnell et al. [29] and our group using PolyA+ RNAs from proliferating and differentiating C2C12 cells ( Fig. 1a ). After Cufflinks assembly, a total of 46,627 transcripts were obtained ( Fig. 1a,b ). After filtering by annotated genes, length, expression and coding potential [30] , a total of 2,413 novel lincRNAs were identified ( Supplementary Data 1 and Fig. 1a,b ), among which 236 are multi-exonic and 3,300 single-exonic. After further annotating each of them with features including K4-K36 domain [12] , EST tag and MyoD binding [31] , a stringent set of 158 lincRNAs ( Fig. 1a,c and Supplementary Data 2 ) were obtained. Further expression analysis revealed that many lincRNAs display a distinct expression pattern with some induced, whereas others repressed, at different time points ( Fig. 1d,e , Supplementary Figs 1a–c and 10 , and Supplementary Data 3 ); a defined lincRNA signature appears to be associated with each stage ( Fig. 1d ). 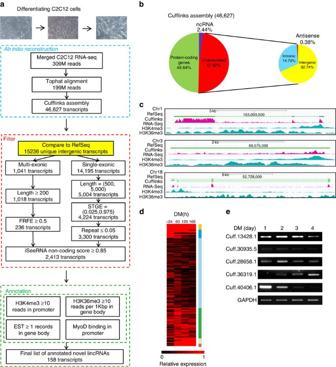Figure 1: Identification of lincRNAs in C2C12 cells. (a) Schematic illustration of an integrative computational pipeline to map and reconstruct, to filter and annotate lincRNAs in C2C12. (b) Annotation of the Cufflinks assembled transcripts (a total of 46627) by Refseq. (c) Genomic snapshots of three novel lincRNA transcripts identified above. (d) Heat map representing the expression profile of novel lincRNAs from proliferating MBs (−24 h) to 168 h in differentiation medium (DM). Colour bars at the right represent gene clusters throughk-means clustering. (e) Validation of five identified lincRNAs by semi-quantitative RT–PCR in differentiating C2C12. Figure 1: Identification of lincRNAs in C2C12 cells. ( a ) Schematic illustration of an integrative computational pipeline to map and reconstruct, to filter and annotate lincRNAs in C2C12. ( b ) Annotation of the Cufflinks assembled transcripts (a total of 46627) by Refseq. ( c ) Genomic snapshots of three novel lincRNA transcripts identified above. ( d ) Heat map representing the expression profile of novel lincRNAs from proliferating MBs (−24 h) to 168 h in differentiation medium (DM). Colour bars at the right represent gene clusters through k -means clustering. ( e ) Validation of five identified lincRNAs by semi-quantitative RT–PCR in differentiating C2C12. Full size image Among all the lincRNAs identified above, a novel transcript initiated upstream of the YY1 gene attracted our attention, owing to its unique location relative to YY1 . The assembled Cufflinks transcript with an estimated size of 793 nt is generated ∼ 2 kb upstream of YY1 ( Fig. 2a ), thus named Linc-YY1 . We cloned it using rapid amplification of complementary DNA ends (RACE), which led to a 1,173-nt transcript possessing a polyadenylation site ( Fig. 2b,c and Supplementary Figs 2a and 10 ); its transcriptional start site is 2,103 bp away from the first exon of YY1 and indeed generated from the opposite strand ( Fig. 2b ). The size was confirmed by northern blotting assay ( Fig. 2d and Supplementary Fig. 10 ). RNA fluorescence in situ hybridization detection revealed it mainly resides in the nuclei of C2C12 MBs and myotubes (MTs), similar to small nuclear transcript U1 ( Fig. 2e and Supplementary Fig. 2b ). This was confirmed by cellular fractionation assay. A high enrichment of Linc-YY1 transcripts was found in nuclear extracts ( Fig. 2f ) together with well-known lncRNAs, Xist, Hotair, Tug1a and U1, and Yam-1 , as we recently showed [11] , was found in both fractions. Consistent with the prediction using our in-house iSeeRNA software [32] ( Supplementary Fig. 3a ) Linc-YY1 is predicted as noncoding by two other publicly available programmes ( Supplementary Fig. 3b–c ), which was confirmed by results from in vitro translation assay ( Supplementary Fig. 3d ). The prediction using RNAfold revealed that it folds into extensive stem–loop structures with the highest thermostability in its middle domain ( Supplementary Fig. 3e ). 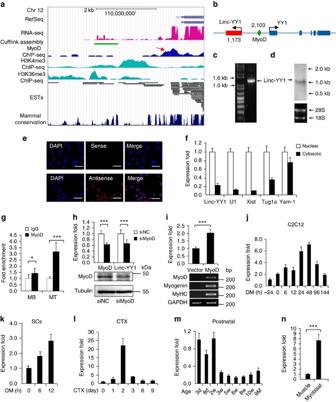Figure 2:De novodiscovery ofLinc-YY1in myogenesis. (a) Genomic snapshot of mouseLinc-YY1generated in Refseq (blue track), H3K4me3, H3K36me3 ChIP-seq (green tracks), MyoD ChIP-seq (blue) and RNA-seq (pink track). (b) Schematic illustration of the genomic location and structure of mouseLinc-YY1relative to theYY1gene. A MyoD binding site at −2,103 is shown as green diamond. Detection of full-lengthLinc-YY1by quantitative RT–PCR (qRT–PCR; 1,173 bp) (c) or northern blotting (d) in C2C12 MBs. (e) Visualization ofLinc-YY1in C2C12 MBs by RNA fluorescencein situhybridization using an antisense probe. As negative control, a sense probe detected no signal. Scale bar, 20 μm. (f) The expression ofLinc-YY1,U1, Xist,Tug1aandYam-1in nuclear or cytosolic fraction of C2C12 MBs. (g) The binding of MyoD on theLinc-YY1promoter by ChIP–PCR. (h) Knockdown of MyoD by siRNA oligos decreasedLinc-YY1expression. (i) Overexpression of MyoD in 10T1/2 cells increasedLinc-YY1expression by qRT–PCR along with the levels ofMyoD,MyogeninandMyHCmRNAs by semi-qRT–PCR. (j) The expression ofLinc-YY1in differentiating C2C12 was detected by qRT–PCR. The expression ofLinc-YY1in (k) differentiating SCs freshly isolated from mouse limb muscles; (l) during CTX-induced regeneration; (m) in muscles of postnatal mice at the indicated ages; (n) in mature mouse muscle or isolated primary MBs. All PCR data were normalized to glyceraldehydes 3-phosphate dehydrogenase (GAPDH) mRNA and represent the average of three independent experiments±s.d. *P<0.05, **P<0.01 and ***P<0.001. Figure 2: De novo discovery of Linc-YY1 in myogenesis. ( a ) Genomic snapshot of mouse Linc-YY1 generated in Refseq (blue track), H3K4me3, H3K36me3 ChIP-seq (green tracks), MyoD ChIP-seq (blue) and RNA-seq (pink track). ( b ) Schematic illustration of the genomic location and structure of mouse Linc-YY1 relative to the YY1 gene. A MyoD binding site at −2,103 is shown as green diamond. Detection of full-length Linc-YY1 by quantitative RT–PCR (qRT–PCR; 1,173 bp) ( c ) or northern blotting ( d ) in C2C12 MBs. ( e ) Visualization of Linc-YY1 in C2C12 MBs by RNA fluorescence in situ hybridization using an antisense probe. As negative control, a sense probe detected no signal. Scale bar, 20 μm. ( f ) The expression of Linc-YY1 , U1, Xist , Tug1a and Yam-1 in nuclear or cytosolic fraction of C2C12 MBs. ( g ) The binding of MyoD on the Linc-YY1 promoter by ChIP–PCR. ( h ) Knockdown of MyoD by siRNA oligos decreased Linc-YY1 expression. ( i ) Overexpression of MyoD in 10T1/2 cells increased Linc-YY1 expression by qRT–PCR along with the levels of MyoD , Myogenin and MyHC mRNAs by semi-qRT–PCR. ( j ) The expression of Linc-YY1 in differentiating C2C12 was detected by qRT–PCR. The expression of Linc-YY1 in ( k ) differentiating SCs freshly isolated from mouse limb muscles; ( l ) during CTX-induced regeneration; ( m ) in muscles of postnatal mice at the indicated ages; ( n ) in mature mouse muscle or isolated primary MBs. All PCR data were normalized to glyceraldehydes 3-phosphate dehydrogenase ( GAPDH ) mRNA and represent the average of three independent experiments±s.d. * P <0.05, ** P <0.01 and *** P <0.001. Full size image If Linc-YY1 is functional during MB differentiation, we reasoned it may be under the regulation of myogenic TF. Indeed, an evident MyoD peak was discovered ∼ 2 kb upstream of the transcription start site (TSS) ( Fig. 2a MyoD chromatin immunoprecipitation sequencing (ChIP-seq) and Fig. 2b ). Results from ChIP–PCR confirmed the association of MyoD on this site, both in MBs and MTs ( Fig. 2g ). Knockdown of MyoD in C2C12 by small interfering RNA (siRNA) oligos decreased Linc-YY1 expression ( Fig. 2h and Supplementary Fig. 10 ), whereas overexpression in mouse embryonic 10T1/2 cells increased its expression ( Fig. 2i and Supplementary Fig. 10 ). To gain more insights, we next assessed its expression in various myogenesis settings. First, during differentiation of C2C12 cells ( Fig. 2j and Supplementary Fig. 4a ), low expression of Linc-YY1 was detected in proliferating MBs at 50% confluence (−24 h). A significant increase was observed when the confluence reached 70–80% (0 day), indicating an induction of Linc-YY1 at the very beginning of myogenic programme induced by cell–cell contact. The expression continuously increased up to 48 h, which was then followed by a gradual decline in the late stages (96 and 144 h); the temporal expression pattern of YY1 gene follows the same profile ( Supplementary Fig. 4b ), indicating their divergent nature in transcription. Consistently, during the differentiation of freshly isolated SCs, Linc-YY1 expression significantly increased in the early stage ( Fig. 2k and Supplementary Fig. 4c ). To further examine its expression dynamics in vivo , we employed a widely used muscle regeneration model in which the injection of cardiotoxin (CTX) results in muscle injury and in turn induces muscle regeneration. After injection with CTX, the tibialis anterior (TA) muscle displays typical degeneration–regeneration process [8] : fibre degeneration and immune cell infiltration are immediately evident within 1 to 2 days, meanwhile SCs start activation and proliferation followed by myogenic differentiation 3–4 days afterwards, newly formed fibres with centrally located nuclei are evident within 5–6 days and muscle architecture is largely restored within 10 days. The expression of Linc-YY1 was found to be rapidly induced starting day 1 and peaked around day 2 ( Fig. 2l and Supplementary Fig. 4d ). Consistently, a higher level of Linc-YY1 was detected in dystrophic muscles of young mdx mice (3 and 5 weeks), which were featured by a pathologically active degeneration–regeneration; this was not observed in limb muscles from normal wild-type mice or older mdx mice (>6 weeks) in which the disease phenotype has subdued ( Supplementary Fig. 4e ). Moreover, high level of Linc-YY1 was observed in limb muscles of newborn mice (age 3 days, 8 days and 2weeks), which displayed active myogenesis but decreased as the neonatal myogenesis ceased after about 2 weeks ( Fig. 2m ). The above results suggested that Linc-YY1 is associated with active myogenesis. Furthermore, when comparing its level in mature skeletal muscle versus SCs, it was highly enriched in the activated SCs or primary MBs isolated from the muscles ( Fig. 2n ), suggesting it is associated with SC activity/function but not muscle tissue homeostasis. Interestingly, it is also broadly expressed in multiple adult tissues with YY1 showing a highly concordant expression pattern ( Supplementary Fig. 4f ). Lastly, by in situ hybridization (ISH), Linc-YY1 transcripts were evidently detectable at E13.5 and E14.5 embryos but were relatively low at other stages ( Supplementary Fig. 5a ); this was confirmed by quantitative reverse-transcriptase PCR (RT–PCR) detection ( Supplementary Fig. 5b ). At E14.5, its expression is evidently high in myotome ( Supplementary Fig. 5a ), suggesting its possible relevance to embryonic myogenesis. Indeed, knockdown of Linc-YY1 by injecting siRNA oligos into the embryos disrupted the myotome formation ( Supplementary Fig. 5c,d ). Collectively, these results led us to believe that Linc-YY1 is a functional molecule in skeletal myogenesis. Linc-YY1 promotes myogenic differentiation of C2C12 cells The early induction of Linc-YY1 during C2C12 differentiation suggested to us that it may be a pro-myogenic factor during MB differentiation. To test this notion, we employed loss- and gain-of-function assays. Successful knockdown of Linc-YY1 ( Supplementary Fig. 6a ) led to a delayed differentiation as assessed by RNA expression of several myogenic markers, Myogenin, MyHC, Tnni2 and α-Actin , and differentiation induced microRNAs, miR-1 and miR-29 ( Fig. 3a ), all of which are known to be direct transcriptional targets of YY1/PRC2 (refs 4 , 5 , 6 , 8 ). Stable knockdown of Linc-YY1 using a short hairpin RNA also delayed the myogenic programme over a course of 6 days ( Fig. 3b and Supplementary Figs 6b and 10 ). Immunofluroscence (IF) staining showed a reduced number of MyHC-positive cells ( Fig. 3c ). Reporter assays using Tnni2, Myogenin and miR-29 luciferase reporters consistently revealed inhibited activities with Linc-YY1 reduction ( Fig. 3d ). These findings confirmed that Linc-YY1 is a pro-myogenic factor during C2C12 differentiation. To strengthen the above findings, Linc-YY1 overexpression was found to accelerate the differentiation of C2C12 cells as assessed using multiple approaches as above ( Fig. 3e–h and Supplementary Fig. 10 ). Lastly, to gain insights into its genome-wide impact, we conducted an RNA-seq analysis to globally characterize Linc-YY1 affected transcriptomic changes. A total of 188 genes were upregulated, whereas only 45 were downregulated by siLinc-YY1 ( Fig. 3i and Supplementary Data 4 ), indicating a predominant gene repressing role for Linc-YY1 . Interestingly, Gene Ontology (GO) analysis revealed that these upregulated genes are enriched for nucleosome and chromatin functions ( Fig. 3j ). Although not significantly enriched as a GO term, expression of several muscle genes was indeed downregulated by siLinc-YY1 ( Supplementary Data 4 ). 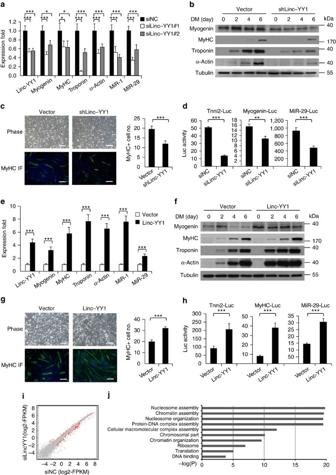Figure 3:Linc-YY1functions to promote C2C12 MB differentiation. (a) Two different siRNA oligos againstLinc-YY1were transfected into C2C12 cells. At 24 h post transfection, the cells were switched to differentiation medium (DM) for 48 h. The expression ofLinc-YY1or the indicated myogenic genes or microRNAs (miRNAs) were then measured. (b) Stable knockdown ofLinc-YY1in C2C12 cells decreased the levels of the indicated proteins during a differentiation course. (c) The above cells were visualized at 2 days in DM. Left: IF staining for MyHC was performed; right: the number of positively stained cells was quantified. (d) C2C12 cells were transfected with siLinc-YY1oligos and the indicated luciferase reporter plasmids. The luciferase activities were measured 48 h after differentiation. (e–h). A Vector orLinc-YY1plasmid was transfected into C2C12 cells and the myogenic assays were performed as ina–d. Overexpression ofLinc-YY1was found to accelerate myogenic differentiation. (i) Knockdown ofLinc-YY1led to significant transcriptomic changes in C2C12 MBs as determined by RNA-seq.XandYaxis represent the log2-based fragments per kilobase of exon per million fragments mapped (FPKM) values for expressed genes in siNC and siLinc-YY1samples, respectively. Differentially expressed genes were shown in red dots. (j) GO analysis of genes that are upregulated in siLinc-YY1compared with siNC. Theyaxis shows the top ten enriched GO terms and thexaxis shows the enrichment significanceP-values. All PCR data were normalized to glyceraldehydes 3-phosphate dehydrogenase (GAPDH) mRNA and represent the average of three independent experiments±s.d. All luciferase data were normalized to Renillia protein and represent the average of three independent experiments±s.d. *P<0.05, **P<0.01 and ***P<0.001. All scale bars, 50 μm. Figure 3: Linc-YY1 functions to promote C2C12 MB differentiation. ( a ) Two different siRNA oligos against Linc-YY1 were transfected into C2C12 cells. At 24 h post transfection, the cells were switched to differentiation medium (DM) for 48 h. The expression of Linc-YY1 or the indicated myogenic genes or microRNAs (miRNAs) were then measured. ( b ) Stable knockdown of Linc-YY1 in C2C12 cells decreased the levels of the indicated proteins during a differentiation course. ( c ) The above cells were visualized at 2 days in DM. Left: IF staining for MyHC was performed; right: the number of positively stained cells was quantified. ( d ) C2C12 cells were transfected with si Linc-YY1 oligos and the indicated luciferase reporter plasmids. The luciferase activities were measured 48 h after differentiation. ( e – h ). A Vector or Linc-YY1 plasmid was transfected into C2C12 cells and the myogenic assays were performed as in a – d . Overexpression of Linc-YY1 was found to accelerate myogenic differentiation. ( i ) Knockdown of Linc-YY1 led to significant transcriptomic changes in C2C12 MBs as determined by RNA-seq. X and Y axis represent the log2-based fragments per kilobase of exon per million fragments mapped (FPKM) values for expressed genes in siNC and si Linc-YY1 samples, respectively. Differentially expressed genes were shown in red dots. ( j ) GO analysis of genes that are upregulated in si Linc-YY1 compared with siNC. The y axis shows the top ten enriched GO terms and the x axis shows the enrichment significance P -values. All PCR data were normalized to glyceraldehydes 3-phosphate dehydrogenase ( GAPDH ) mRNA and represent the average of three independent experiments±s.d. All luciferase data were normalized to Renillia protein and represent the average of three independent experiments±s.d. * P <0.05, ** P <0.01 and *** P <0.001. All scale bars, 50 μm. Full size image Linc-YY1 functions in SCs and muscle regeneration To extend our findings in C2C12 cells to a more physiologically relevant setting, we tested the function of Linc-YY1 in freshly isolated SCs. In keeping with its pro-myogenic function in C2C12 cells, knockdown of Linc-YY1 by siRNA oligos impaired myogenic differentiation of the cells, whereas overexpression of Linc-YY1 improved their differentiation ( Fig. 4a,b ). These findings were further confirmed on SCs associated with freshly isolated single myofibres, which serve as an excellent ex vivo model. Knockdown or overexpression of Linc-YY1 on the myofibres led to an inhibition or enhancement of SC activities as assessed by both Myogenin and Pax7 staining ( Fig. 4c,d ). Furthermore, to extend these in vitro findings to in vivo muscle formation, we explored the function of Linc-YY1 in CTX-induced muscle regeneration. Treatment of regenerating muscles with si Linc-YY1 oligos following a scheme as described before [33] ( Fig. 4e ) led to downregulation of Pax7, MyoD, Myogenin and embryonic-MyHC (e-MyHC , a marker for regenerating fibres) at both messenger RNA and protein levels ( Fig. 4f,g and Supplementary Fig. 10 ). In addition, the expression of the regeneration-associated miR-1 and miR-29 (refs 5 , 8 ) was also inhibited ( Fig. 4f ). Consistently, IF staining on the muscle sections revealed a decreased number of cells positively stained by Pax7, MyoD and Myogenin, and the number of newly formed fibres with centrally localized nuclei and the fibre size were also decreased by si Linc-YY1 injection ( Fig. 4h and Supplementary Fig. 6c,d ). These findings implied that depletion of Linc-YY1 suppressed muscle regeneration. Altogether, our results suggested that Linc-YY1 is a functional pro-myogenic factor in muscle SCs and during muscle regeneration in vivo . 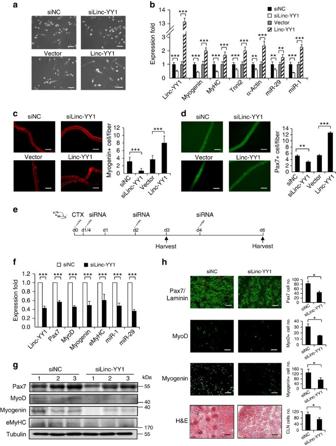Figure 4:Linc-YY1is a pro-myogenic factor in SCs and muscle regeneration. (a,b)siLinc-YY1or control oligos were transfected into the freshly isolated SCs to knockdown ofLinc-YY1; Vector orLinc-YY1expression plasmid was transfected into the cells to overexpressLinc-YY1. The gene expression was measured 48 h post transfection. (c,d) Single fibres were isolated from mouse limbs and transfected withsiLinc-YY1orLinc-YY1plasmid, to knock down or overexpressLinc-YY1. IF staining for Myogenin and Pax7 was performed 48 h post transfection. (e) Injection scheme for siNC or siLinc-YY1oligos into CTX injured muscles.N=4 mice for each group.Linc-YY1siRNA injection decreased the levels of the indicated RNAs (f) and proteins (g) at day 6 in three representative mice. (h) IF staining for Pax7, Laminin, MyoD and Myogenin was performed on the above injected muscles at day 3. Positively stained cells were quantified. The muscles were also stained with haematoxylin and eosin at day 6. Fibres with centrally localized nuclei (CLN) were quantified. All PCR data were normalized to glyceraldehydes 3-phosphate dehydrogenase (GAPDH) mRNA and represent the average of three independent experiments±s.d. *P<0.05, **P<0.01 and ***P<0.001. All scale bars, 50 μm. Figure 4: Linc-YY1 is a pro-myogenic factor in SCs and muscle regeneration. ( a , b ) siLinc-YY1 or control oligos were transfected into the freshly isolated SCs to knockdown of Linc-YY1 ; Vector or Linc-YY1 expression plasmid was transfected into the cells to overexpress Linc-YY1 . The gene expression was measured 48 h post transfection. ( c , d ) Single fibres were isolated from mouse limbs and transfected with siLinc-YY1 or Linc-YY1 plasmid, to knock down or overexpress Linc-YY1 . IF staining for Myogenin and Pax7 was performed 48 h post transfection. ( e ) Injection scheme for siNC or si Linc-YY1 oligos into CTX injured muscles. N =4 mice for each group. Linc-YY1 siRNA injection decreased the levels of the indicated RNAs ( f ) and proteins ( g ) at day 6 in three representative mice. ( h ) IF staining for Pax7, Laminin, MyoD and Myogenin was performed on the above injected muscles at day 3. Positively stained cells were quantified. The muscles were also stained with haematoxylin and eosin at day 6. Fibres with centrally localized nuclei (CLN) were quantified. All PCR data were normalized to glyceraldehydes 3-phosphate dehydrogenase ( GAPDH ) mRNA and represent the average of three independent experiments±s.d. * P <0.05, ** P <0.01 and *** P <0.001. All scale bars, 50 μm. Full size image Linc-YY1 promotes myogenesis through regulating YY1 activity Next, we probed into the molecular mechanisms underlying the promoting role of Linc-YY1 in myogenesis. Considering cis regulation of their neighbouring genes has been a favourable mode of action for many well-studied lincRNAs including Xist [34] , HOTTIP [21] and Mistral [35] , we tested first the possibility of Linc-YY1 directly regulating YY1 transcription. Manipulation of Linc-YY1 levels by siRNA or overexpression in C2C12 cells resulted in only a modest change of YY1 mRNA or protein ( Supplementary Figs 7a,b and 10 , and Fig. 5a ); it also did not modulate the levels of PRC2 components. However, as it inhibited the transcription of several known direct targets of YY1, such as MyHC, Tnni2, miR-1 and miR-29 ( Figs 3 and 4 ), all of which are co-regulated by PRC2, we speculated that instead of acting in cis , Linc-YY1 could bind with YY1/PRC2 complex to antagonize its transcriptional activity on these muscle loci in trans . This would also explain why ectopic expression of Linc-YY1 could promote the expression of these target genes and elicit the pro-myogenic phenotype ( Fig. 4a–d ). To test this hypothesis, we performed RNA immunoprecipitation (RIP) assay [36] ( Supplementary Fig. 7c ). Expectedly, IP of YY1, Ezh2 or Embryonic ectoderm development (Eed) from proliferating C2C12 MBs at 80–90% confluence (MBs) or early differentiating MTs pulled down significant amount of Linc-YY1 ( Fig. 5b and Supplementary Figs 7d and 10 ). To further determine the specific interacting protein partner, we performed RNA pull-down assay ( Supplementary Fig. 7e ) from native non-cross-linked cell lysates using biotinylated in vitro -synthesized RNA. Contrary to our original thought that Linc-YY1 may bind to PRC2 similar to many other lincRNAs, the full-length Linc-YY1 retrieved no Ezh2 or Suz12 and very low level of Eed; however, it retrieved a substantial amount of YY1 ( Fig. 5c and Supplementary Fig. 10 ), suggesting that Linc-YY1 specifically binds with YY1. To further map the binding domain, a series of deletion mutants of Linc-YY1 were generated and the middle domain that retained nculeotides 386–851 pulled down YY1 with almost equal efficiency as the full-length fragment; 5′ (1–414) or 3′ (832–1173) domain, on the other hand, could not retrieve much YY1. It suggested that the middle domain most probably contains functional structures, which is in accordance with its high thermostability ( Supplementary Fig. 3e ). Indeed, at the functional level overexpression of the middle domain, but not the other two domains, recapitulated the full-length function, leading to the increase of YY1/PRC2 target gene expression ( Fig. 5d ). To map the YY1 domain that interacts with Linc-YY1 , various fragments of YY1 were expressed in C2C12 and the domain of 174–200 appears to be necessary and sufficient for retrieving Linc-YY1 ( Fig. 5e and Supplementary Fig. 10 ). 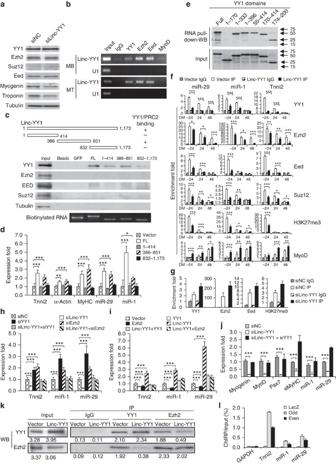Figure 5:Linc-YY1regulates YY1/PRC2 transcriptional activity through binding to YY1. (a) Expression of YY1, Ezh2, Eed and Suz12 proteins was measured in C2C12 cells transfected with control or siLinc-YY1oligos and differentiated for 48 h. (b) RIP assay was performed using antibodies against YY1, Ezh2, EED or MyoD. The retrievedLinc-YY1transcripts were detected by RT–PCR.U1transcripts were used as a negative control. (c) Biotin-labelled full-length (fl) or the middle domain ofLinc-YY1transcripts were used to retrieve YY1, Ezh2, Eed or Suz12 proteins. (d) The plasmid expressing various domains or the fl domain ofLinc-YY1was transfected into C2C12 cells and the gene expression was measured 48 h post differentiation. (e) Various HA-tagged YY1 domains were expressed in C2C12 MBs (input), pulled down by biotinylatedLinc-YY1transcripts and examined by western blotting (WB). (f) Vector orLinc-YY1was expressed in C2C12 cells and ChIP–PCR was performed to detect the enrichment of the indicated proteins onmiR-29a/b1,miR-1-1andTnni2promoter at differentiation medium (DM) −24, 24 and 48 h. (g)Linc-YY1oligos were injected into CTX injured muscles to knock downLinc-YY1and the enrichment of YY1/PRC2 and H3K27me3 on Tnni2 promoter was detected by ChIP–PCR. (h) The indicated siRNA oligos were transfected into C2C12 and the gene expression was measured 48 h post differentiation. (i) The indicated expression plasmids were transfected into C2C12 cells and the gene expression was measured 48 h post differentiation. (j) The indicated siRNA oligos were injected into the CTX-injuried muscles and the gene expression was measured 6 days post injection. (k) Vector orLinc-YY1was transfected into the C2C12 cells and lysates harvested 48 h post transfection for co-immunoprecipitation assay to detect the interaction between YY1 and Ezh2. (l) Chromatin isolation by RNA purification (ChIRP) assay was performed using even and odd antisense oligos tilinglinc-YY1and a significant amount of genomic DNAs corresponding toTnni2, miR-1andmiR-29promoters but not in glyceraldehydes 3-phosphate dehydrogenase (GAPDH) locus was retrieved. LacZ ChIRP retrieved no signal. All PCR data were normalized toGAPDHmRNA and represent the average of three independent experiments±s.d. *P<0.05, **P<0.01 and ***P<0.001. Figure 5: Linc-YY1 regulates YY1/PRC2 transcriptional activity through binding to YY1. ( a ) Expression of YY1, Ezh2, Eed and Suz12 proteins was measured in C2C12 cells transfected with control or si Linc-YY1 oligos and differentiated for 48 h. ( b ) RIP assay was performed using antibodies against YY1, Ezh2, EED or MyoD. The retrieved Linc-YY1 transcripts were detected by RT–PCR. U1 transcripts were used as a negative control. ( c ) Biotin-labelled full-length (fl) or the middle domain of Linc-YY1 transcripts were used to retrieve YY1, Ezh2, Eed or Suz12 proteins. ( d ) The plasmid expressing various domains or the fl domain of Linc-YY1 was transfected into C2C12 cells and the gene expression was measured 48 h post differentiation. ( e ) Various HA-tagged YY1 domains were expressed in C2C12 MBs (input), pulled down by biotinylated Linc-YY1 transcripts and examined by western blotting (WB). ( f ) Vector or Linc-YY1 was expressed in C2C12 cells and ChIP–PCR was performed to detect the enrichment of the indicated proteins on miR-29a/b1 , miR-1-1 and Tnni2 promoter at differentiation medium (DM) −24, 24 and 48 h. ( g ) Linc-YY1 oligos were injected into CTX injured muscles to knock down Linc-YY1 and the enrichment of YY1/PRC2 and H3K27me3 on Tnni2 promoter was detected by ChIP–PCR. ( h ) The indicated siRNA oligos were transfected into C2C12 and the gene expression was measured 48 h post differentiation. ( i ) The indicated expression plasmids were transfected into C2C12 cells and the gene expression was measured 48 h post differentiation. ( j ) The indicated siRNA oligos were injected into the CTX-injuried muscles and the gene expression was measured 6 days post injection. ( k ) Vector or Linc-YY1 was transfected into the C2C12 cells and lysates harvested 48 h post transfection for co-immunoprecipitation assay to detect the interaction between YY1 and Ezh2. ( l ) Chromatin isolation by RNA purification (ChIRP) assay was performed using even and odd antisense oligos tiling linc-YY1 and a significant amount of genomic DNAs corresponding to Tnni2, miR-1 and miR-29 promoters but not in glyceraldehydes 3-phosphate dehydrogenase ( GAPDH ) locus was retrieved. LacZ ChIRP retrieved no signal. All PCR data were normalized to GAPDH mRNA and represent the average of three independent experiments±s.d. * P <0.05, ** P <0.01 and *** P <0.001. Full size image The above results led us to further hypothesize that Linc-YY1 binds to YY1/PRC2 repressive complex on early differentiation, leading to its eviction from chromatins and subsequent de-repression of the previously known YY1/PRC2 co-regulated targets. To test this notion, we performed ChIP assays using chromatins from Vector- or Linc-YY1 -overexpressing C2C12 cells collected at -24, 24 and 48 h of differentiation. The association of YY1/PRC2 with several previously known target promoters including miR-29a/b1, miR-1-1 and Tnni2 was examined by ChIP–PCR. As expected ( Fig. 5f and Supplementary Fig. 7f ), the enrichment of YY1/PRC2 was very high in proliferating C2C12 MBs and gradually declined during the myogenic differentiation from day 1 to day 2. Indeed, the overexpression of Linc-YY1 caused concurrent loss of YY1, Ezh2, Eed and Suz12 binding at all three time points on all the three promoters examined. These results suggested that ectopic expression of Linc-YY1 could evict YY1/PRC2 complex from the known target promoters, confirming its in trans function. Additional ChIP for H3K27me3 indicated a concurrent loss on the target promoters. Interestingly, the loss of YY1/PRC2 binding is accompanied by a gain of MyoD binding, which is in keeping with our previous finding that MyoD-activating complex replaces YY1/PRC2 to activate these target genes [6] . Therefore, Linc-YY1 titrates away YY1/PRC2 binding on muscle loci in trans . Furthermore, when tested in the CTX-induced regenerating muscles, knockdown of Linc-YY1 by siRNA oligo injection increased the occupancy of YY1/PRC2 on their target promoters ( Fig. 5g and Supplementary Fig. 7g ), suggesting this mechanism also applied in vivo . To further elucidate whether the Linc-YY1 function on these targets is dependent on YY1/PRC2, we performed functional rescue assays. Knockdown of YY1 or Ezh2 successfully rescued the inhibitory effect of si Linc-YY1 on the target gene expression ( Fig. 5h ), wherease overexpression suppressed the pro-myogenic effect of Linc-YY1 expression ( Fig. 5i ). Furthermore, in regenerating muscles knockdown of YY1 also overcome the inhibitory effect of si Linc-YY1 ( Fig. 5j ), suggesting to us that Linc-YY1 effects on these promoters are largely through regulating YY1/PRC2 activity. To further answer the question how Linc-YY1 removes YY1/PRC2 complex from the target promoters, we sought to test whether Linc-YY1 binding to YY1 destabilizes its association with PRC2. Indeed, we found that expression of Linc-YY1 hampered the interaction between endogenous YY1 and Ezh2 proteins using co-immunoprecipitation assay ( Fig. 5k and Supplementary Figs 7h and 10 ). Furthermore, using chromatin isolation by RNA purification (ChIRP) assay [37] with both odd and even tiling oligos against Linc-YY1 , we were able to specifically retrieve substantial amount of endogenous Linc-YY1 transcripts from the target loci ( Fig. 5l and Supplementary Fig. 7i–k ). Altogether, the above findings provided compelling evidence to support the notion that on the known target genes Linc-YY1 functions through antagonizing YY1/PCR2 transcriptional activities in trans . The above findings demonstrated one important mechanism of Linc-YY1 action, that is, its regulation of YY1/PRC2 as a complex on the known targets. Considering our recent genome-wide mapping revealed the Ezh2 independent aspect of YY1 function, we performed ChIP-seq for YY1/PRC2 in the above C2C12 MBs ( Supplementary Data 5 ), aiming to explore additional mechanisms of gene regulation. Interestingly, 43% of YY1-binding peaks were lost in Linc-YY1 -expressing cells but the total peak number was significantly increased ( Fig. 6a ), suggesting that Linc-YY1 expression not only caused eviction on some loci but gain of occupancy on many other loci ( Supplementary Fig. 8a ). With regard to Ezh2 binding, a similar number of total peaks were identified in Vector- versus Linc-YY1 -expressing cells but very little overlapping was found between the two data sets, suggesting a genome-wide shift of Ezh2 binding caused by Linc-YY1 , which was also observed for H3K27me3 occupancy. Eed binding, on the other hand, is very different in a sense that a dramatic loss of occupancy (95%) was induced by Linc-YY1 , although the total or nuclear level of Eed protein was not significantly decreased by Linc-YY1 ( Fig. 5a and Supplementary Fig. 8b ). 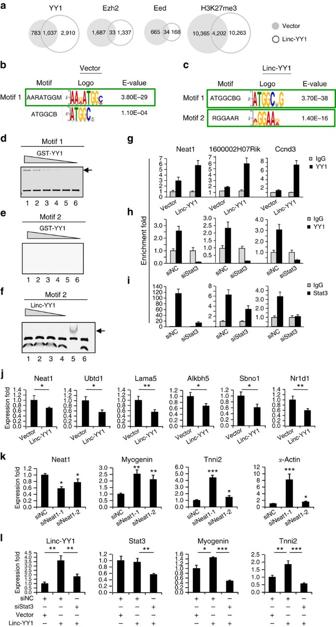Figure 6: Effect ofLinc-YY1overexpression on YY1 and PRC2 genome-wide binding. (a) Venn diagram showing the overlapping between the ChIP-seq data sets from the above Vector orLinc-YY1-expressed cells. Ectopic expression ofLinc-YY1affected genome-wide binding of YY1/PRC2 and H3K27me3. (b,c) Motif analysis of the YY1-binding peaks from vector andLinc-YY1groups. An YY1 canonical binding sequence was identified as the most significantly enriched motif (Motif 1) in Vector peaks. A binding motif (Motif 2) was identified inLinc-YY1peaks as the second most enriched motif. (d) electrophoretic mobility shift (EMSA) assay was used to detect the direct association between Motif 1 and purified GST-YY1 protein at a serial titration (Lane 1–6: GST-YY1 400, 200, 100, 50, 25 and 0 nM). Arrow denotes the formation of the DNA/protein-binding complex. (e) No direct binding between Motif 2 and GST-YY1 protein was detected by EMSA assay (Lane 1–6: GST-YY1 400, 200, 100, 50, 25 and 0 nM). (f) No binding between Motif 2 and GST-YY1 was detected with the addition ofin vitrotranscribedLinc-YY1RNAs at a serial titration (Lane 1–4:Linc-YY112, 6, 3 and 0 ng μl−1+GST-YY1 400 nM; Lane 5: GST-YY1 400 nM with Motif 1 as positive control; Lane 6: GST only with Motif 2 as negative control). (g) YY1 ChIP was performed in Vector- orLinc-YY1-transfected cells, to confirm theLinc-YY1-induced YY1 binding to Motif 2 on three selected target loci,Neat1,1600002H07RikandCcnd3. (h) The above binding was abolished by knocking down ofStat3using an siRNA oligo. (i) Stat3 binding was also diminished by the above siStat3 treatment. (j)Linc-YY1overexpression led to repression of the YY1/Stat3 co-bound target genes,Neat1,Ubtd1,Lama5,Alkbh5,Sbno1,Nr1d1. (k) Knockdown ofNeat1by two different siRNA oligos accelerated myogenic differentiation as assessed by the increased expression ofMyogenin,Tnni2andα-Actin. (l) Knockdown ofStat3by siRNA oligos abolished the pro-myogenic effect ofLinc-YY1as assessed by the expression ofMyogeninandTnni2. *P<0.05, **P<0.01 and ***P<0.001. Figure 6: Effect of Linc-YY1 overexpression on YY1 and PRC2 genome-wide binding. ( a ) Venn diagram showing the overlapping between the ChIP-seq data sets from the above Vector or Linc-YY1 -expressed cells. Ectopic expression of Linc-YY1 affected genome-wide binding of YY1/PRC2 and H3K27me3. ( b , c ) Motif analysis of the YY1-binding peaks from vector and Linc-YY1 groups. An YY1 canonical binding sequence was identified as the most significantly enriched motif (Motif 1) in Vector peaks. A binding motif (Motif 2) was identified in Linc-YY1 peaks as the second most enriched motif. ( d ) electrophoretic mobility shift (EMSA) assay was used to detect the direct association between Motif 1 and purified GST-YY1 protein at a serial titration (Lane 1–6: GST-YY1 400, 200, 100, 50, 25 and 0 nM). Arrow denotes the formation of the DNA/protein-binding complex. ( e ) No direct binding between Motif 2 and GST-YY1 protein was detected by EMSA assay (Lane 1–6: GST-YY1 400, 200, 100, 50, 25 and 0 nM). ( f ) No binding between Motif 2 and GST-YY1 was detected with the addition of in vitro transcribed Linc-YY1 RNAs at a serial titration (Lane 1–4: Linc-YY1 12, 6, 3 and 0 ng μl −1 +GST-YY1 400 nM; Lane 5: GST-YY1 400 nM with Motif 1 as positive control; Lane 6: GST only with Motif 2 as negative control). ( g ) YY1 ChIP was performed in Vector- or Linc-YY1 -transfected cells, to confirm the Linc-YY1 -induced YY1 binding to Motif 2 on three selected target loci, Neat1 , 1600002H07Rik and Ccnd3 . ( h ) The above binding was abolished by knocking down of Stat3 using an siRNA oligo. ( i ) Stat3 binding was also diminished by the above siStat3 treatment. ( j ) Linc-YY1 overexpression led to repression of the YY1/Stat3 co-bound target genes, Neat1 , Ubtd1 , Lama5 , Alkbh5 , Sbno1 , Nr1d1 . ( k ) Knockdown of Neat1 by two different siRNA oligos accelerated myogenic differentiation as assessed by the increased expression of Myogenin , Tnni2 and α-Actin . ( l ) Knockdown of Stat3 by siRNA oligos abolished the pro-myogenic effect of Linc-YY1 as assessed by the expression of Myogenin and Tnni2 . * P <0.05, ** P <0.01 and *** P <0.001. Full size image The above results suggested Linc-YY1 expression exerted very different impact on YY1 and PRC2, somehow reflecting their genome-wide independency as we recently reported. To further explore additional aspects of Linc-YY1 regulation of YY1 activity, we performed in-depth analysis of the above sequencing data. Using de novo motif analysis, we found that YY1 predominantly bound to its canonical binding motif, AANATGG, in Vector control cells ( Fig. 6b , Motif 1). The peaks containing this motif remained unchanged on Linc-YY1 overexpression, ( Fig. 6c , Motif 1); however, another motif, RGGAAR, appeared as the second most significantly enriched sequence ( Fig. 6c , Motif 2); it suggested that Linc-YY1 overexpression may have induced YY1-binding affinity towards this previously unknown motif. Using electrophoretic mobility shift assays, however, we did not detect a direct association between purified GST-YY1 protein and Motif 2 on addition of Linc-YY1 transcripts ( Fig. 6d–f ). Therefore, it is likely to be that the binding towards this motif is mediated indirectly through another TF, as YY1 is well known to cooperate with many co-factors in regulating gene expression. Interestingly, Motif 2 highly resembles binding sequence for Stat3. By ChIP–PCR, the Linc-YY1 -induced YY1 binding on selective loci was confirmed ( Fig. 6g ) and knockdown of Stat3 ( Supplementary Fig. 8c ) abolished the binding ( Fig. 6h,i ). Interestingly, many of these Stat3/YY1-bound target genes such as Neat1 , Ubtb1 , Lama5 , Alkbh5 , Sbno1 and Nr1d1 were repressed by Linc-YY1 overexpression ( Fig. 6j ), implying that Linc-YY1 may repress their expression through inducing YY1/Stat3 binding. Functionally, knocking down Neat1 promoted the differentiation as shown in Fig. 6k . Together, the above result suggested in addition to activating genes through evicting YY1/PRC2, Linc-YY1 could also promote myogenesis through Stat3/YY1-mediated gene repression. Consistent with the thinking, we found knockdown of Stat3 abolished the pro-myogenic effect of Linc-YY1 ( Fig. 6l ). Altogether, the above results thus confirmed our thought that globally Linc-YY1 possesses other functions additional to evicting YY1/PRC2 from the known target promoters. Linc-YY1 function is conserved in human MBs Although conservation is not a general feature for lincRNAs [28] , a modest level of mammal conservation was observed on Linc-YY1 locus ( Fig. 2a ). Mining the GENCODE annotation, an lncRNA transcript, RP11-63812, was discovered upstream of human YY1 gene locus ( Fig. 7a,b ). Evidence of expression of this transcript in many human cells (for example, GM12878, K562 and Embryonic Stem cells) was also found through mining ENCODE RNA-seq data. The expression of h Linc-YY1 during myogenic differentiation mirrored that of m Linc-YY1 in C2C12 cells: a gradual induction during early differentiation followed by a decline ( Fig. 7c ). Furthermore, knockdown of hLinc-YY1 in human MBs caused impairment of myogenic differentiation ( Fig. 7d,e ), which is analogous to the effect of depleting mouse Linc-YY1 in C2C12 cells. Similarly, hLinc-YY1 was found to be associated with YY1 in human MBs and MTs ( Fig. 7f ), and knockdown of hLinc-YY1 stabilized YY1 association with target muscle loci ( Fig. 7g ). Together, these results suggested to us that the function of Linc-YY1 is conserved in mouse and human myogenesis. 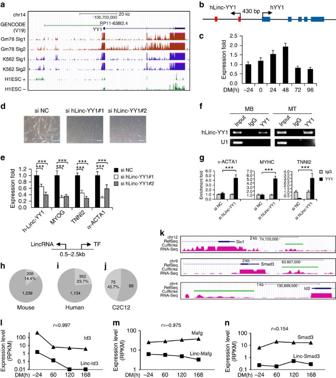Figure 7:Linc-YY1function is conserved in human and lincRNA/TF association is a general phenomenon. (a) Snapshot of the lncRNA associated with humanYY1promoter. RP11-63812.4 was identified from the GENCODE annotation (version 19). Evidence of expression is shown in GM12878 cells (two replicates), K562 cells (two replicates) and H1ESC cells (plus or minus strand signals) by RNA-seq reads from ENCODE. (b) The genomic location and structure of human (h)Linc-YY1430 bp away from humanYY1gene. (c) The expression levels ofhLincYY1during human MB differentiation. Knockdown of hLinc-YY1by siRNA oligos in human MBs inhibited the differentiation as assessed by (d) the cell morphology and (e) the expression of myogenic markers,MYOG,TNNI2andα-ACTA1. Scale bar, 50 μm. (f) YY1 bound to hLinc-YY1but not U1 in human MBs or MTs as revealed by RIP assay. (g) By ChIP–PCR assays, knockdown of hLinc-YY1by siRNA oligos in human MBs increased the enrichment of YY1 on three target muscle loci,α-ACTA1,MYHCandTNNI2. (h,i) TF-LincRNA pairs were identified in mouse and human using ENSEMBL gene annotation. (j) A total of 164 TF-lincRNA pairs were identified in C2C12 cells. Seventy-five of them showed no correlation, whereas 89 displayed positive or negative correlation in their expressions during C2C12 differentiation. (k) Snapshots of lincRNAs associated withSix1,Smad3andId3in C2C12 cells. (l) Correlated expression ofId3and its associated LincRNA,Linc-Id3during C2C12 differentiation course. Pearson’sr=0.997. (m) Anti-correlated expression ofMafgandLinc-Mafg. Pearson’s r=−0.975. (n) No correlation was identified in the expression ofSmad3andLinc-Smad3. Pearson’sr=0.154. Figure 7: Linc-YY1 function is conserved in human and lincRNA/TF association is a general phenomenon. ( a ) Snapshot of the lncRNA associated with human YY1 promoter. RP11-63812.4 was identified from the GENCODE annotation (version 19). Evidence of expression is shown in GM12878 cells (two replicates), K562 cells (two replicates) and H1ESC cells (plus or minus strand signals) by RNA-seq reads from ENCODE. ( b ) The genomic location and structure of human (h) Linc-YY1 430 bp away from human YY1 gene. ( c ) The expression levels of hLincYY1 during human MB differentiation. Knockdown of h Linc-YY1 by siRNA oligos in human MBs inhibited the differentiation as assessed by ( d ) the cell morphology and ( e ) the expression of myogenic markers, MYOG , TNNI2 and α-ACTA1 . Scale bar, 50 μm. ( f ) YY1 bound to h Linc-YY1 but not U1 in human MBs or MTs as revealed by RIP assay. ( g ) By ChIP–PCR assays, knockdown of h Linc-YY1 by siRNA oligos in human MBs increased the enrichment of YY1 on three target muscle loci, α-ACTA1 , MYHC and TNNI2 . ( h , i ) TF-LincRNA pairs were identified in mouse and human using ENSEMBL gene annotation. ( j ) A total of 164 TF-lincRNA pairs were identified in C2C12 cells. Seventy-five of them showed no correlation, whereas 89 displayed positive or negative correlation in their expressions during C2C12 differentiation. ( k ) Snapshots of lincRNAs associated with Six1 , Smad3 and Id3 in C2C12 cells. ( l ) Correlated expression of Id3 and its associated LincRNA, Linc-Id3 during C2C12 differentiation course. Pearson’s r =0.997. ( m ) Anti-correlated expression of Mafg and Linc-Mafg . Pearson’s r=−0.975. ( n ) No correlation was identified in the expression of Smad3 and Linc-Smad3 . Pearson’s r =0.154. Full size image Transcription of lincRNA/TF pair is a general phenomenon The discovery of Linc-YY1 /YY1 regulation led us to ask whether divergently transcribed lincRNAs regulating TF transcriptional activity is a general phenomenon. We inspected 1,447 mouse TFs for possible evidence of divergent transcription using ENSEMBL gene annotation (version 70 for hg19 and version 67 for mm9). We limited our search to a region of −0.5 to −2.5 kb upstream, to exclude transcripts overlapping with TF or those originating more distantly (>2.5 kb). Indeed, the presence of at least one divergent transcript was discovered in a high portion of TFs (14.4%; Fig. 7h and Supplementary Data 6 ). This was also observed in human: 23.7% of 1,486 TFs have divergently transcribed lincRNAs on their promoter regions ( Fig. 7i and Supplementary Data 6 ). We further examined the expression correlation of 164 TF/lincRNA pairs identified from our C2C12 RNA-seq data ( Fig. 7j,k and Supplementary Fig. 9 ) reasoning that correlated pairs have higher chance to regulate each other’s expression in cis . Eighty-nine of the pairs displayed either a positive or a negative correlation on the basis of a Pearson’s correlation analysis ( Fig. 7l,m and Supplementary Data 7 ); nevertheless, a large portion (45.7%) showed discordant expression ( Fig. 7n and Supplementary Data 7 ), raising the possibility that these lincRNAs may instead regulate the TF activity in trans . Through combining several RNA-seq data sets from differentiating C2C12 cells, our study provides a catalogue of novel lincRNAs in muscle cells, which serves as a valuable resource for future functional exploration. It is worth pointing out that by using the uniquely designed Sebnif 30 software, we were able to identify a strikingly large number of single-exonic lincRNAs (3,300 single exonic versus 236 multi-exonic), indicating the prevalence of single-exonic lincRNAs. More reports clearly demonstrate that bona fide single-exonic lncRNAs are as functional as multi-exonic ones; therefore, the common practice of omitting single-exonic transcripts to simplify the identification pipeline may lead to an incomplete catalogue of lincRNAs. Despite the rapidly increasing number of lincRNAs functionally investigated so far, research of lincRNA in myogenesis is still at its infancy with a handful being characterized to date [11] , [38] , [39] , [40] . Our study provides a comprehensive characterization of Linc-YY1 functionally and mechanistically. The findings from this study demonstrate its important regulatory function during the process of MB differentiation into MTs. In addition, it could also regulate other aspects of SC activities. In particular, as it is known that YY1/PRC2 regulates Pax7 expression through binding to its promoter [41] , it is possible that Linc-YY1 could regulate SC activation/proliferation through modulating Pax7. Indeed, we observed the downregulation of Pax7 on Linc-YY1 knockdown in both single fibre-associated SCs and regenerating muscles ( Fig. 4 ). On top of its role in the muscle, as YY1 is a ubiquitously expressed TF, which plays vital roles in numerous biological settings, Linc-YY1 may have an even broader role in regulating YY1 function beyond myogenesis. For example, in ES cells where YY1/PRC2 plays an essential role in regulating differentiation [42] , [43] , Linc-YY1 may exert its roles through modulating YY1/PRC2 activities. Unlike many LincRNAs, which are not evolutionally conserved, a human Linc-YY1 was also found to be associated with human YY1 gene and functions to promote myogenesis through associating and modulating YY1 activity. Thus, Linc-YY1 appears to be evolutionally conserved in its function despite lacking conservation in its primary sequence. This is consistent with the speculation that it is probably the secondary structure of lincRNAs that dictates their function [13] . With the deletion mapping we were able to determine that the middle part of Linc-YY1 (386–851) comprising stable stem–loop structures seems sufficient to bind YY1 and is highly functional in terms of promoting myogenesis ( Fig. 5 ). In the future it will be interesting to study its secondary structure and search for its protein-binding domains to gain a greater understanding of structure-to-function relationships. With regard to the molecular mechanisms, we have focused on its regulation of YY1 activity. In particular, we uncovered how it regulates the transcriptional activity of YY1/PRC2 complex on several previously known target genes ( Fig. 8 ). Its mode of action is unique in several ways. First, it does not seem to physically interact with any member of PRC2 similar to many other lincRNAs; instead, it binds to YY1 directly. This is not an utter surprise considering that YY1 has long been known to possess high-affinity RNA-binding activity [44] . More recently, YY1 has been shown to tether lncRNA, Xist, to the inactive X chromosome nucleation centre through direct association with C repeat region of Xist, thus qualifying as a bivalent TF, which binds to both RNA and DNA [45] . It is also interesting to point out that unlike other PRC2-associated lincRNAs, which target or guide PRC2 to genomic sites causing gene silencing, Linc-YY1 removes YY1/PRC2 to cause the known target gene activation. In contrast to what is known about TF/epigenetic factor recruitment, less is known in terms of how they are removed to ensure timely regulation of gene expression. It is generally explained through the degradation of the proteins, which may require changes in signalling cascades. Our studies revealed a mechanism through which TF/epigenetic regulators can be removed effectively before their degradation. Biochemically, it is still unclear how Linc-YY1 association with YY1 destabilizes the YY1/PRC2 complex. It is possible that Linc-YY1 binding disrupts YY1 association with DNA element, but our results demonstrated that it is more likely to3 be that Linc-YY1 binding disrupts the association between YY1 and Ezh2. As Linc-YY1 does not seem to bind the REPO domain of YY1, which is known to be necessary for Polycomb group protein recruitment [46] , it will be interesting to explore how this disruption occurs in the future. Considering the importance of having these known target genes silenced in the MB cells, Linc-YY1 regulation of YY1/PRC2 activity provides a mechanistic explanation for its pivotal role in myogenesis; nonetheless, our recent study also revealed that YY1/PRC2 co-binding is not observed genome wide [11] , raising the interesting possibility that Linc-YY1 could also regulate PRC2-independent aspect of YY1 function. Indeed, our ChIP-seq analysis in the Linc-YY1 -overexpressing cells showed that Linc-YY1 expression exerted very different effect on YY1 and PRC2 member binding globally. Linc-YY1 not only evicted YY1 from some loci but also re-directed it to other loci, partly through its interaction with Stat3. Preliminary investigation showed that Linc-YY1 possibly represses the expression on at least some of these YY1/Stat3 bound loci such as a well-known Neat1 , raising an interesting scenario that the pro-myogenic function of Linc-YY1 could also be mediated through YY1/Stat3 interaction ( Fig. 8 ). However, we argue that the focus of the study should be the YY1/PRC2-dependent mechanism; future efforts will be devoted to dissect other diverse functional mechanisms through which Linc-YY1 regulates myogenesis. 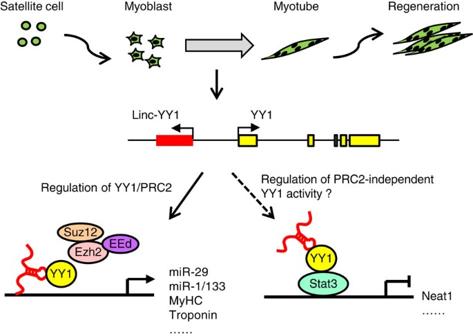Figure 8: A model ofLinc-YY1functions in myogenesis. The model depicts the role of theLinc-YY1in MB differentiation. When differentiation starts,Linc-YY1(red colour) is transcribed concurrently from upstream of theYY1gene (yellow). On the known YY1/PRC2 target promoters,miR-29,miR-1,MyHC,Troponinand so on,Linc-YY1binds to YY1, causing the dissociation and eviction of YY1/PRC2 complex from target promoters, which then leads to the activation of target genes.Linc-YY1could also exert its function through regulating PRC2-independent function of YY1, for example,Linc-YY1may recruit YY1 to Stat3-bound loci and repressNeat1or other targets. Other aspects ofLinc-YY1regulation remain unclear and will be explored in the future. Figure 8: A model of Linc-YY1 functions in myogenesis. The model depicts the role of the Linc-YY1 in MB differentiation. When differentiation starts, Linc-YY1 (red colour) is transcribed concurrently from upstream of the YY1 gene (yellow). On the known YY1/PRC2 target promoters, miR-29 , miR-1 , MyHC , Troponin and so on, Linc-YY1 binds to YY1, causing the dissociation and eviction of YY1/PRC2 complex from target promoters, which then leads to the activation of target genes. Linc-YY1 could also exert its function through regulating PRC2-independent function of YY1, for example, Linc-YY1 may recruit YY1 to Stat3-bound loci and repress Neat1 or other targets. Other aspects of Linc-YY1 regulation remain unclear and will be explored in the future. Full size image Several genome-wide studies have suggested that promoters of protein-coding genes are origins of ncRNA transcription [27] . In particular, our study showed that many TFs generate divergent lincRNAs from their promoters. This is in line with a recent report showing divergent transcription is associated with promoters of transcriptional regulators [24] . This phenomenon supports the notion that lincRNAs are integrated components of transcriptional regulatory networks through their regulation of TFs either in cis or in trans . Direct regulation on TF expression in cis seems a more favourable mode due to the physical proximity and would require low number of lincRNA molecules. Nevertheless, in trans modulation of TF transcriptional activity allows direct regulation on a broader array of targets. This seems to be common at least during myogenic differentiation, as many TF/LincRNA pairs from C2C12 cells displayed no correlation in their expressions. Being generated from the same promoter allows for the concurrent appearance of LincRNAs with the TF, benefiting their action in concert. Yet, it remains to be determined how the lincRNA moves within nucleus and specifically binds with the TF to guide it to or remove it from the trans targets. One possibility is that the TF binds the same motifs on DNA and the lincRNA, but this was not found to be the case in YY1–Xist association [45] . It is also likely to be that the interaction could occur in the cytosol where many lincRNAs are found. The search for the answers will probably bring future surprises. Cells Mouse C2C12 MBs (CRL-1772) were obtained from ATCC and cultured in DMEM medium supplemented with 10% fetal bovine serum (FBS), 2 mM L -glutamine, 100 U ml −1 penicillin and 100 μg of streptomycin at 37 °C in 5% CO 2 . For myogenic differentiation, cells were seeded in 60- or 100-mm plates and shifted to DMEM containing 2% horse serum (HS) when 90% confluence. Primary MBs were isolated from ∼ 1-week-old mice muscles as described before [8] , [47] . Briefly, total hind limb muscles (three to six mice per group) were digested with 5 mg ml −1 type IV collagenase (Life Technologies, Carlsbad, CA) and 1.4 mg ml −1 dispase II (Life Technologies) for 0.5 h, and cell suspensions were filtered through 70 and 40 μM cell strainer, respectively, then pre-plated for an hour. Non-adherent cells were centrifuged and cultured on Gelatin-coated plates (Iwaki, Japan) in F10 medium (Life Technologies) supplemented with 20% FBS and basic fibroblast growth factor (Life Technologies, 25 ng ml −1 ). After removing fibroblasts by pre-plating, primary MB cells were cultured in F10/DMEM medium (1:1) supplemented with 20% FBS and basic fibroblast growth factor. Human skeletal MBs (HSkM-S, Invitrogen) were maintained in F10 medium supplemented with 20% FBS and shifted to DMEM containing 2% HS for differentiation. 10T1/2 cells (CCL-226) were cultured in DMEM supplemented with 10% FBS and induced to myogenic differentiation after MyoD transfection by shifting to DMEM containing 2% HS. Transfections and infections Transient transfection of cells with siRNA oligos or DNA plasmids was performed on 60 or 100-mm dishes with Lipofectamine 2000 reagent as suggested by the manufacturer (Invitrogen). For luciferase experiments, C2C12 and primary MBs were transfected in 12-well plates. Cell extracts were prepared and luciferase activity was monitored as previously described [4] using Dual-Luciferase kit (Promega). To generate C2C12 cells stably expressing Linc-YY1, a Linc-YY1-expressing plasmid (4 μg) was transfected into C2C12 cells using Lipofectamin 2000 (Invitrogen). Thirty-six hours after transfection, cells were placed in 400 μg ml −1 G418 (Invitrogen) for stable selection. Stable clones were pooled together after ∼ 2 weeks selection. To generate C2C12 cells with Linc-YY1 stably knocked down, an empty pSIREN-RetroQ Retroviral vector (Clontech) or pSIREN/shLnc-YY1 along with the packaging plasmid (pSIREN Helper) were transfected into HEK293T cells. Forty-eight hours after transfection, supernatant was harvested from these cells and titrited. Approximately 1 × 10 9 virus particles were used to transduce C2C12 cells, which were subsequently placed in 2 μg ml −1 puromycin for selection. Stable clones were pooled together after 1 week selection. Single fibre isolation and use Two of extensor digitorum longus muscles were excised from C57BL/6 mice and digested in 1 ml of DMEM medium containing 500 U ml −1 Collagenase II, 10% HS, 1% Pen/Strep at 37 °C with gentle agitation for 75 min. The digestion solution is then transferred into 20 ml of pre-warmed DMEM containing 10% HS, 1% Pen/Strep, 20 mM HEPES pH 7.3 in HS-precoated 100 mm Petri dish. Single fibres were liberated by gently triturating the digested extensor digitorum longus muscles against the edge of Petri dish using a fire polished Pasteur pipet with wide tip. Once around 100 fibres have fallen off, the dishes were placed back to the incubator. Individual, healthy (non-shrinking) fibres were transferred to a new HS-coated 100-mm dish using the HS-coated P1000 tips every 15–25 min and the transfer was repeated three times to remove debris and the interstitial cells from fibres. Finally, 50 single fibres were transferred to each 35 mm dish with 1 ml of HamF10 medium containing 10% HS, 0.05% chick embryo extract and cultured in suspension. Transfection was performed at the same day. siRNA (50 pmol) or 2 μg plasmid is mixed with 1 μl Lipofectamine 2000 in 50 μl Opti-MEM I and incubated for 20 min before adding to myofibres and incubated at 37 °C for overnight. In general, every 24 h 50% of the medium was replaced with Ham’s F10 medium with 20% FBS. For differentiation, 24 h after transfection, 50% of the medium was replaced with DMEM containing 2% HS and incubated for 3 days. For IF staining, fibres were fixed with 2% paraformaldehyde in medium and stained using anti-Pax7 or anti-Myogenenin antibodies. The number of Pax7 or Myogenin-positive cells was quantified from at least 20 fibres. This procedure was adapted from ref. 48 . Cell fractionation Cells were harvested after tripsinization and washed with PBS twice. Cell pellet was then resuspended in RSB buffer (10 mM Tris pH 7.4, 10 mM NaCl, 3 mM MgCl 2 ) and incubated on ice for 3 min followed by centrifugation at 4 °C. The pellet was then resuspended in RSBG40 buffer (10 mM Tris pH 7.4, 10 mM NaCl, 3 mM MgCl 2 , 10% glycerol, 0.5% Noidet P-40, 0.5 mM dithiothretol (DTT) and 100 U ml −1 rRNasin) followed by centrifugation. The supernatant was transferred to a new tube as cytoplasmic fraction; the pellet was resuspended in RSGB40 buffer with one-tenth volume of detergent (3.3% sodium deoxycholate and 6.6% Tween 40) followed by centrifugation. The supernatant was saved as cytoplasmic fraction. The pellet was used as nuclear fraction. RNAs were extracted from both fractions using Trizol. This procedure was adapted from ref. 6 . Rapid amplification of cDNA end SMARTer RACE cDNA Amplification Kit (Clontech) was used according to the manufacturer’s instructions. Briefly, to generate 5′-RACE-Ready cDNAs, 1 μg total RNAs extracted from C2C12 MBs were reverse transcribed using 5′-CDS Primer A, SMARTer IIA oligo and SMARTScribe Reverse Transcriptase. The subsequent PCR amplification was carried out using a gene-specific reverse primer and a Universal Primer Mixture from the kit. 3′-RACE-Ready cDNAs were obtained by using 3′-CDS Primer A. The primer sequences can be found in Supplementary Data 8 . DNA constructs An YY1 expression plasmid was a gift from Y. Shi (Harvard University) [6] . A miR-29-promoter luciferase reporter was created before and 200 ng was used per transfection [5] . Renilla luciferase reporter was obtained from Promega and used as per the manufacturer’s protocol. Replication-deficient retroviral-based expression plasmids pSIREN-RetroQ vector was obtained from System Biosciences (SBI). The pSIREN/sh Linc-YY1 -expressing plasmid was constructed by annealing synthetic oligos containing an siRNA sequence against Linc-YY1 to BamHI and EcoRI cloning sites according to the manufacturer’s instruction (Clontech). Full-length 5′ (1–414 bp), middle (386–856 bp) and 3′ (832–1173, bp) domains of Linc-YY1 were PCR amplified and cloned by T–A cloning into modified pBluescript KS(+), while enhanced green fluorescent protein ( EGFP ) was cloned into the XbaI site of pcDNA3.1(+) for in vitro transcription. To generate mammalian expression vectors for full-length Linc-YY1 , it was PCR amplified and cloned into NheI and KpnI sites of pcDNA3.1(+). Expressing plasmids for 5′ or middle domain of Linc-YY1 were cloned using BamHI and XhoI sites, while for the 3′ domain were cloned with XhoI and XbaI sites from their corresponding T–A constructs. Primers used for cloning can be found in Supplementary Data 8 . In vitro transcription For producing sense transcripts of the above full-length and deletion mutant fragments, in vitro transcription was performed using MAXIscript T7/T3 kit (Ambion) after linearization of the plasmids. Oligonucleotides The following 19-nucleotide duplex siRNAs were used: mouse YY1 (#1, 5′-GAACUCACCUCCUGAUUAU-3′; #2, 5′-CCAGAAUGAAGCCAAGAAA-3′); mouse Ezh2 (5′-GAGGAAGACUUCCGAAUAA-3′); mouse Linc-YY1 (#1, 5′-GCAUAUUAUCACACAUCUA-3′; #2, 5′-CCUGAAACCAACACAUAUA-3′); human Linc-YY1 (#1, 5′-GCGAAAGUCUGCAGCUUCA-3′; #2, 5′-CCGUGAAGAACAAGCAACU-3′) or scrambled oligos were obtained from Ribobio. In each case, 50 μM oligos were used for transient transfections into cells or injection into mouse muscles. The sequences of oligos can be found in Supplementary Data 8 . RT–PCR and northern blotting analysis Total RNAs from cells were extracted using TRIzol reagent (Life Technologies) according to the manufacturer’s instructions and cDNAs were prepared using M-MLV (Moloney murine leukemia virus) Reverse Transcriptase (Life Technologies) and Oligo(dT)20 primer. Expression of mRNA analysis was performed with SYBR Green Master Mix (Life Technologies) as described on an ABI PRISM 7900HT Sequence Detection System (Life Technologies) using glyceraldehydes 3-phosphate dehydrogenase for normalization [50] . For northern blotting analysis, the DNA probe was labelled with dCTP[α-32P] (PerkinElmer) using RadPrime DNA Labeling System (Invitrogen). RNA fluorescence in situ hybridization DNA probe with size of 50–500 bp was prepared using Vysis nick translation kit (catalogue number 32–801300 and Spectrum-green dUTP) for direct labelling. Cells grown on coverslip were rinsed briefly in PBS and then fixed in 4% freshly prepared formaldehyde in PBS (pH 7.4) for 15 min at room temperature (RT). The cells were then permeabilized in PBS containing 0.2–0.5% Triton X-100 and 2 mM VRC (New England Biolabs Inc., USA) on ice for 10 min and washed with PBS 3 × 10 min and 2 × SSC for 10 min before hybridization. Two microlitres of probe (100–500 ng) and yeast transfer RNA (20 μg) were then redissolved in 10 μl formamide (Ambion), which was denatured at 90 °C for 10 min and immediately chilled on ice for 5 min. The 20 μl hybridization cocktail containing the denatured probe, 10% Dextran sulfate and RNase inhibitor (Invitrogen) in 2 × SSC was added to each coverslip for hybridization at 37 °C overnight (12–16 h) in a humidified chamber. After a series of wash with SSC solution, the cells were counter stained with 4,6-diamidino-2-phenylindole for observation. This procedure was adapted from ref. 11 . RNA pull-down assay Biotinylated RNAs were prepared using MAXIscript T7/T3 In vitro transcription kit (Ambion) and Biotin RNA labelling Mix (Roche). The above RNAs were denatured at 90 °C for 2 min and then renatured with RNA structure buffer (Ambion) at RT for 20 min. C2C12 cell pellets (5 × 10 6 ) were treated with 20% nuclear isolation buffer (1.28 M sucrose, 40 mM Tris-HCl pH 7.5, 20 mM MgCl 2 , 4% Triton X-100) with 1 × Complete Protease Inhibitor Cocktail (PIC, Roche). Nuclei were collected by 2,500 g centrifugation for 15 min. Nuclear pellet was resuspended in 1 ml RIP buffer (150 mM KCl, 25 mM Tris pH 7.4, 0.5 mM DTT, 0.5% NP40, 1 mM phenylmethyl sulfonyl fluoride and 1 × PIC) and sonicated with three cycles (30 s interval, 30 s sonication) using Bioruptor (Diagenode). After centrifugation at 13,000 r.p.m. for 10 min to remove nuclear membrane and debris, 1 mg of C 2 C 12 nuclear extract was then mixed with 3 μg of renatured RNA respectively and incubated at RT for 1 h. Thirty microlitres of washed streptavidin agarose beads (Invitrogen) were added to each pull-down reaction and further incubated at RT for 1 h. Beads were pelleted and washed for five times in Handee spin columns (Pierce) using RIP buffer. The resulting beads were boiled in western blotting loading buffer to retrieve the proteins, which were then detected by standard western blotting technique. RIP assay C2C12 cells were cross-linked with 1% formaldehyde and collected for lysis by radioimmunoprecipitation assay (RIPA) buffer (50 mM Tris pH 7.4, 150 mM NaCl, 1 mM EDTA, 0.1% SDS, 1% NP-40 and 0.5% sodium deoxycholate, 0.5 mM DTT, 1 mM phenylmethyl sulfonyl fluoride, 1 × Proteinase inhibitor cocktail and 1% RNaseOut) [36] . The lysate was incubated with specific antibodies or normal IgG control for overnight. The RNA/protein complex was recovered with protein G Dynabeads and washed with RIPA buffer several times. After reverse cross-link with proteinase K at 45 °C for 45 min, RNA was recovered with Trizol and analysed by RT–PCR. Antibody-based assays For western blotting analyses, total cell extracts were prepared in RIPA buffer [33] , [51] . The following dilutions were used for each antibody: myogenin (Santa Cruz Biotechnology; 1:2,000), MyoD (Santa Cruz Biotechnology; 1:2,000), α-Skeletal Actin (Sigma; 1:2,000), Troponin (Sigma; 1:2,000), MyHC (Sigma; 1:2,000), YY1 (Santa Cruz Biotechnology; 1:2,000), Ezh2 (Active Motif, 1:2,000), Suz12 (Abcam, 1:2,000), Eed (Millipore, 1:2,000), α-Tubulin (Sigma; 1:5,000), Pax 7 (Developmental Studies Hybridoma Bank; 1:2,000), eMyHC (Leica, 1:2,000) and glyceraldehydes 3-phosphate dehydrogenase (Santa Cruz Biotechnology; 1:5,000). Densimetric quantification of the western bands was performed using the Quantity One software (Bio-Rad). Immunofluorescence on cultured cells and single fibres was performed using the following antibodies: MyHC (Sigma; 1:350), Myogenin (Santa Cruz Biotechnology; 1:350), MyoD (Santa Cruz Biotechnology; 1:350) and Pax 7 (Developmental Studies Hybridoma Bank; 1:2,000). Frozen muscle sections were prepared by immersion in isopentene in liquid nitrogen [33] , [51] . Immunoflurescence staining on frozen muscle sections was performed using the following antibodies: MyoD (Santa Cruz, 1:100); Myogenin (Santa Cruz, 1:100) and Pax7 (DSHB, 1:100). Haematoxylin and eosin staining was performed on frozen muscle sections (5 μm) [33] , [51] . Quantification of number of fibres with centrally located nuclei and IF positively stained cells was performed from a minimum of 20 randomly chosen fields, from 5–6 sections throughout the length of the muscle in 4–6 per group. All fluorescent images were captured with an Axioplan 2 imaging universal microscope (Zeiss, Germany). All samples were imaged with the × 20 or × 40 objective lens. Co-immunoprecipitation assay Ten micrograms of Normal IgG (Santa Cruz Biotechnology), antibodies against YY1 (Santa Cruz Biotechnology) or Ezh2 (Active Motif) were cross-linked to 50 μl (bed volume) of Protein A/G PLUS-Agarose (Santa Cruz Biotechnology) by dimethyl pimelimidate (Sigma). C2C12 cells were cross-linked with 200 μg ml −1 of 3,3′-Dithiodipropionic acid di(N-hydroxysuccinimide ester) (Sigma) for 20 min and then harvested and lysed in RIPA buffer (25 mM HEPES pH 7.4, 1% Nonidet P-40, 0.1% SDS, 0.5% sodium deoxycholate, 1 × PIC). The antibody-conjugated beads were incubated with 500 μg of the above cell lysate overnight at 4 °C with rotation. After extensive washing with RIPA buffer, the bound proteins were eluted by boiling in 20 μl of 2 × sample buffer (125 mM Tris-HCl pH 6.8, with 4% SDS, 20% (v/v) glycerol) and subjected to western blotting analysis. ChIP assay ChIP assays using chromatins from C2C12 MBs or MTs were performed using 5 μg of antibodies against YY1 (Santa Cruz Biotechnology), Ezh2 (Active Motif), trimethyl-histone H3-K27 (Millipore), Suz12 (Abcam), Eed (Millipore), MyoD (Santa Cruz Biotechnology) or isotype IgG (Santa Cruz Biotechnology) used as a negative control. Genomic DNA pellets were resuspended in 20 μl of water. Quantitative RT–PCR was performed with 1 μl of immunoprecipitated material with SYBR Green Master Mix (Bio-Rad Laboratories). Relative enrichment is calculated as the amount of amplified DNA normalized to input and relative to values obtained after normal IgG immunoprecipitation, which were set as 1. Primers used are listed in Supplementary Data 8 . In vivo ChIP was performed following a modified protocol described in ref. 52 . Briefly, muscles were collected, finely minced and fixed in 2 × volume of PBS containing 1% formaldehyde for 10 min at RT. A volume (1/20) of 2.5 M glycine was then added to quench formaldehyde. The fixed tissues was suspended in 10 ml of Lysis buffer 1 (50 mM HEPES-KOH pH 7.5, 140 mM NaCl, 1 mM EDTA, 10% glycerol, 0.5% NP-40, 0.25% Triton X-100, 1 × protease inhibitors) and homogenized with IKA T10 basic homogenizer (ScienceLab). The resulting homogenate was then rocked at 4 °C on platform rocker for 10 min followed by centrifugation at 1,350 g for 5 min at 4 °C. The pellet was then resuspended in 10 ml of Lysis Buffer 2 (10 mM Tris-HCl pH 8.0, 200 mM NaCl, 1 mM EDTA, 0.5 mM EGTA, 1 × protease inhibitors) and proceeded to ChIP as described above and in refs 8 , 33 . ISH in mouse embryos and muscles Inbred Institute for Cancer Research pregnant mice were obtained from the animal house and embryos at different developmental stages (gestational day 6.5 (E6.5)–E17.5) were prepared under a stereomicroscope (Leica, Germany). For ISH, preparations were kept in PBS (0.1% diethyl pyrocarbonate), and extra embryonic tissue was removed. Whole embryos and corresponding controls were fixed in 4% formaldehyde, dehydrated in graded methanol solutions. The fixed embryos were dehydrated in graded ethanol/xylene mixtures and then embedded in paraffin. Sagittal sections of the embryos at 5-μm thickness were prepared and stored at RT before in situ hybridization. Suitable antisense riboprobes were prepared by transcription of a pBluescript KS(+) plasmid containing a 700-bp-long 5′-’RACE-cloned Linc-YY1 fragment using T3 RNA polymerase (Ambion), to incorporate digoxigenin-11-UTP (Roche). The hybridization signal was developed by anti-digoxigenin alkaline phosphatase. For ISH detection of Linc-YY1 on regenerating muscles, the frozen muscle sections were prepared by immersion in isopentene in liquid nitrogen [33] , [51] and the ISH detection was performed as above. Animal studies All animal experiments were performed in strict adherence to the guidelines for experimentation with laboratory animals set in institutions. mdx (C57BL/10 ScSn DMDmdx) were purchased from the Jackson Laboratory (Bar Harbor, ME). C57B/L and mdx mice were housed in the animal facility of the Chinese University of Hong Kong under conventional conditions with constant temperature and humidity, and fed a standard diet. Animal experimentation was approved by the Chinese University of Hong Kong Animal Experimentation Ethics Committee (Ref. No. 10/027/MIS). For CTX injection, ∼ 7-week-old male mice were injected with 50 μl of CTX at 10 μg ml −1 into the TA muscles. Oligos were prepared by pre-incubating 2 μM of siRNA oligos with Lipofectamine 2000 for 15 min and injections were made in a final volume of 50 μl in OPTI-EM (GIBCO). Mice were killed and TA muscles were harvested at designated days, and total RNAs and proteins were extracted for real-time RT–PCR and western blotting analyses. For IF staining of MyoD, Myogenin and Pax7, TA muscles were collected at day 3, while at day 6 TA muscles were collected for haematoxylin and eosin staining. RNA-sequencing Preparation of RNA-seq libraries for sequencing on the Illumina platforms was carried out using the RNA-Seq Sample Preparation Kit (catalogue number RS-930-1001) according to the manufacturer’s standard protocol. Briefly, purified RNA was fragmented via incubation for 5 min at 94 °C with the Illumina-supplied fragmentation buffer. The first strand of cDNA was next synthesized by reverse transcription using random oligo primers. Second-strand synthesis was conducted by incubation with RNase H and DNA polymerase I. The resulting double-stranded DNA fragments were subsequently end-repaired and A-nucleotide overhangs were added by incubation with Taq Klenow lacking exonuclease activity. After the attachment of anchor sequences, fragments were PCR amplified using Illumina-supplied primers and loaded onto the Hiseq 2000 or GAIIx flow cell. DNA clusters were generated with an Illumina cluster station with Paired-End Cluster Generation Kit v2 (Illumina), followed by 50 (or 36) × 2 cycles of sequencing on sequencer with Sequencing Kit v3 (Illumina). Genome Analyzer Sequencing Control Software (SCS) v2.5, which could perform real-time image analysis and base calling, was used to carry out the image processing and base calling during the chemistry and imaging cycles of a sequencing run. The default parameters within the data analysis software (SCS v2.5) from Illumina were used to filter poor-quality reads. In the default setting, a read would be removed if a chastity of <0.6 is observed on two or more bases among the first 25 bases. To evaluate the expression profiles of novel lincRNAs, Cufflinks (version 2.0.2) was used to quantitate the gene expression at each time point. The lincRNAs were then clustered by Cluster 3.0 (version 1.50) software ( http://bonsai.hgc.jp/~mdehoon/software/cluster/ ) [53] using k -means ( k =6) with Euclidean distance as the similarity metric. To detect the differentially expressed genes between siNC- and siLinc-YY1-transfected C2C12 cells, the raw RNA-seq data were first preprocessed (adapter trimming and duplicate removing using in-house programmes) and then aligned to the reference genome (UCSC mm9) using Tophat (version 2.0.4), during which procedure the UCSC gene annotation file downloaded from Cufflinks website ( http://cole-trapnell-lab.github.io/cufflinks/igenome_table/index.html ) was used (the ‘-G’ option of Tophat). Cuffdiff (version 2.0.4) was then applied on the aligned data set, to determine differentially expressed genes with a ‘significant’ status. The GO analysis of the differentially expressed genes was performed using DAVID ( http://david.abcc.ncifcrf.gov/ ). ChIP-sequencing To construct ChIP-seq library, the purified DNA (10 ng) was end-repaired and A-nucleotide overhangs were added by incubation with the Taq Klenow fragment lacking exonuclease activity [11] . After the attachment of anchor sequences, fragments were PCR amplified using Illumina-supplied primers. The purified DNA library products were evaluated using Bioanalyzer (Agilent) and SYBR quantitative PCR and diluted to 10 nM for sequencing on Illumina GAIIx or Hiseq 2000 sequencer (pair end with 36 or 50 bp). A data analysis pipeline SCS v2.5 (Illumina) was employed to perform the initial bioinformatics analysis including base calling and converting the results into raw reads in FASTQ format. Peak defining The sequenced reads were mapped to the mouse reference genome (UCSC mm9) using SOAP2 (ref. 54 ). The alignment was performed, allowing the maximum of two mismatches and keeping only the uniquely aligned reads. The protein DNA-binding peaks (sites) were identified using Model-based Analysis for ChIP-seq (MACS, version 1.4.2) [55] with IgG control sample as the background. During the peak calling, the P -value cutoff was set to under 10 −5 for all ChIP-seq experiments. RNA secondary structure analysis Secondary structure analysis was performed using Vienna RNAfold server ( http://rna.tbi.univie.ac.at/cgi-bin/RNAfold.cgi ), to do minimum free energy structure analysis. Statistical analysis Statistical significance was assessed by the Student’s t -test. (* P <0.5, ** P <0.01 and *** P <0.001). Accession codes : RNA-seq/ChIP-seq data have been deposited in GEO under the following Accession codes: GSE74049, GSM 1908734, GSM 1908735, GSM 1908736, GSM 1908737, GSM 1908738, GSM 1908739, GSM 1908740, GSM 1908741, GSM 1908742, GSM 1908743, GSM 1908744, GSM 1908745 and GSM 1908746. How to cite this article: Zhou, L. et al. Linc-YY1 promotes myogenic differentiation and muscle regeneration through an interaction with the transcription factor YY1. Nat. Commun. 6:10026 doi: 10.1038/ncomms10026 (2015).